Quantum phases with differing computational power The observation that concepts from quantum information has generated many alternative indicators of quantum phase transitions hints that quantum phase transitions possess operational significance with respect to the processing of quantum information. Yet, studies on whether such transitions lead to quantum phases that differ in their capacity to process information remain limited. Here we show that there exist quantum phase transitions that cause a distinct qualitative change in our ability to simulate certain quantum systems under perturbation of an external field by local operations and classical communication. In particular, we show that in certain quantum phases of the XY model, adiabatic perturbations of the external magnetic field can be simulated by local spin operations, whereas the resulting effect within other phases results in coherent non-local interactions. We discuss the potential implications to adiabatic quantum computation, where a computational advantage exists only when adiabatic perturbation results in coherent multi-body interactions. The study of quantum phase transitions has greatly benefited from developments in quantum information theory [1] , [2] . We know, for example, that the extremum points of entanglement and other related correlations coincide with phase transition points [3] , [4] , [5] , [6] , [7] , and that different phases may feature differing fidelity between neighbouring states [8] , [9] , [10] , [11] , [12] , [13] . These observations have helped pioneer many alternative indicators of phase transitions, allowing the tools of quantum information science to be harnessed in the analysis of quantum many-body systems [1] , [2] . The reverse, however, remains understudied. If the concepts of quantum information processing have such relevance to the study of quantum phase transitions, one would expect that systems undergoing quantum phase transition would also exhibit different operational properties from the perspective of information processing. Yet, there remains little insight on how such relations are applied to quantum information and computation. In this paper, we demonstrate using the XY model that different quantum phases have distinct operational significance with respect to quantum information processing. We reveal that the differential local convertibility of ground states undergoes distinct qualitative change at points of phase transition. By differential local convertibility of ground states, we refer to the following ( Fig. 1 ): a given physical system with an adjustable external parameter g is partitioned into two parties, Alice and Bob. Each party is limited to local operations on their subsystems (which we call A and B ) and classical inter-party communication, i.e., local operations and classical communication (LOCC). The question is: can the effect on the ground state caused by adiabatic perturbation of g be achieved through LOCC by Alice and Bob? Differential local convertibility of ground states is significant. Should LOCC operations between Alice and Bob be capable of simulating a particular physical process, then such a process is of limited computational power, that is, it is incapable of generating any quantum coherence between A and B . 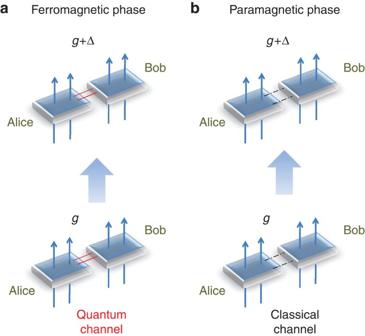Figure 1: Differential local convertibility illustration. Alice and Bob control the two bipartitions of a physical system whose ground state depends on a Hamiltonian that can be varied via some external parameterg. In one phase (a), the conversion from one ground state |G(g)〉 to another |G(g+Δ)〉 requires a quantum channel between Alice and Bob, that is, coherent interactions between the two partitions are required. We say that this phase has no local convertibility. After phase transition (b), Alice and Bob are able to convert |G(g)〉 to |G(g+Δ)〉 via only local operations and classical communications, and local convertibility becomes possible. If Δ→0, local convertibility becomes differential local convertibility. This implies that it is impossible to completely simulate the adiabatic evolution of the ground state with respect togby LOCC in one quantum phase and possible in the other phase. Figure 1: Differential local convertibility illustration. Alice and Bob control the two bipartitions of a physical system whose ground state depends on a Hamiltonian that can be varied via some external parameter g . In one phase ( a ), the conversion from one ground state | G ( g )〉 to another | G ( g +Δ)〉 requires a quantum channel between Alice and Bob, that is, coherent interactions between the two partitions are required. We say that this phase has no local convertibility. After phase transition ( b ), Alice and Bob are able to convert | G ( g )〉 to | G ( g +Δ)〉 via only local operations and classical communications, and local convertibility becomes possible. If Δ→0, local convertibility becomes differential local convertibility. This implies that it is impossible to completely simulate the adiabatic evolution of the ground state with respect to g by LOCC in one quantum phase and possible in the other phase. Full size image We make use of the most powerful notion of differential local convertibility, that of LOCC operations together with assisted entanglement [14] , [15] . Given some infinitesimal Δ, let | G ( g )〉 AB and | G ( g +Δ)〉 AB be the ground states of the given system when the external parameter is set to be g and g +Δ, respectively. The necessary and sufficient conditions for local conversion between | G ( g )〉 AB and | G ( g +Δ)〉 AB is given by S α ( g )≥ S α ( g +Δ) for all α , where is the Rényi entropy with parameter α , ρ A ( g ) is the reduced density matrix of | G ( g )〉 AB with respect to Alice's subsystem and { λ i } are the eigenvalues of ρ A ( g ) in decreasing order [16] , [17] , [18] . Thus, if the Rényi entropies of two states intercept for some α , they cannot convert to each other by LOCC even in the presence of ancillary entanglement [19] . In the Δ→0 + limit, we may instead examine the sign of ∂ g S α ( g ) for all α . If ∂ g S α ( g ) does not change sign, the effect of an infinitesimal increase of g results in global shift in S α ( g ), with no intersection between S α ( g +Δ) and S α ( g ). Otherwise, an intersection must exist. Transverse field Ising model Before we consider the general XY model, we highlight key ideas on the transverse Ising model, which has the Hamiltonian where σ k , for k = x , y , z , are the usual Pauli matrices, and periodic boundary conditions are assumed. The transverse Ising model is one of the simplest models that has a phase transition, therefore it often serves as a test bed for applying new ideas and methods to quantum phase transitions. Osterloh et al . [3] have previously shown that the derivative of the concurrence is a indicator of the phase transition. Nielsen et al . [4] have also studied concurrence between two spins at zero or finite temperature Recently, the Ising chain with frustration has been realized in the experiment [20] . The transverse Ising model features two different quantum phases, separated by a critical point at g =1. When g <1, the system resides in the ferromagnetic (symmetric) phase. It is ordered, with non-zero order parameter 〈 σ x 〉, that breaks the phase flip symmetry When g >1, the system resides in the symmetric paramagnetic (symmetry broken) phase, such that 〈 σ x 〉=0. There is systematic qualitative difference in the computational power afforded by perturbation of g within these two differing phases. In the paramagnetic phase, ∂ g S α ( g ) is negative for all α , hence increasing the external magnetic field that can be simulated by LOCC. In the ferromagnetic phase, ∂ g S α ( g ) changes signs for certain α. Thus, the ground states are not locally convertible, and perturbing the magnetic field in either direction results in fundamentally non-local quantum effects. This result is afforded by the study of how Rényi entropy within the system behaves. From equation (1), we see that Rényi entropy contains all knowledge of { λ i } [21] . For large vanishes when λ i is small, and larger eigenvalues dominate. In the limit where α →∞, all but the largest eigenvalue λ 1 may be neglected such that In contrast, for small values of α , smaller eigenvalues become as important as their larger counterparts. In the α →0 + limit, the Rényi entropy approaches to the logarithm of the rank for the reduced density matrix, that is, the number of non-zero eigenvalues. This observation motivates study of the eigenvalue spectrum. In systems of finite size ( Fig. 2a ), the largest eigenvalue monotonically increases while the second monotonically decreases for all g . All the other eigenvalues λ k exhibit a maximum at some point g k . From the scaling analysis ( Fig. 2b and c ), we see that as we increase the size of the system, g k →1 for all k . Thus, in the thermodynamic limit, λ k exhibits a maximum at the critical point of g =1 for all k ≥3. Knowledge of this behaviour gives intuition to our claim. 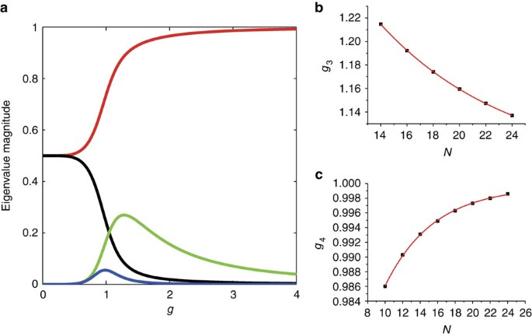Figure 2: The largest four eigenvalues and the scaling analysis. (a) The four largest eigenvalues of transverse Ising ground state forN=10 case. The red line represents the largest eigenvalueλ1and the black line is the second oneλ2. Note that we have artificially magnifiedλ3(green) andλ4(blue) by ten times for the sake of clarity as each subsequent eigenvalue is approximately one order smaller than its predecessor. (b) The scaling behaviours of the maximal points of the third eigenvalue. WhenN→∞, the maximum points approach to the critical point with certain acceptable error. The black dots are the data and the red curves are the exponential fit of these data. The maximum point for the third eigenvalue(c) The maximum point for the fourth eigenvalueThe maximum points of smaller eigenvalues have similar behaviour. Figure 2: The largest four eigenvalues and the scaling analysis. ( a ) The four largest eigenvalues of transverse Ising ground state for N =10 case. The red line represents the largest eigenvalue λ 1 and the black line is the second one λ 2 . Note that we have artificially magnified λ 3 (green) and λ 4 (blue) by ten times for the sake of clarity as each subsequent eigenvalue is approximately one order smaller than its predecessor. ( b ) The scaling behaviours of the maximal points of the third eigenvalue. When N →∞, the maximum points approach to the critical point with certain acceptable error. The black dots are the data and the red curves are the exponential fit of these data. The maximum point for the third eigenvalue ( c ) The maximum point for the fourth eigenvalue The maximum points of smaller eigenvalues have similar behaviour. Full size image In the ferromagnetic phase, that is, 0< g <1, ∂ g S α ( g ) takes on different signs for different α . When α →0 + , S α tends to the logarithm of the effective rank. From Fig. 2, we see that all but the two largest eigenvalues increase with g , resulting in an increase of effective rank. Thus ∂ g S α ( g )>0 for small α . In contrast, when α →∞, As λ 1 increases with g ( Fig. 2 ), ∂ g S α ( g )<0 for large α . Therefore, there is no differential local convertibility in the ordered phase. In the paramagnetic phase, that is, g >1, calculation yields that ∂ g S α ( g ) is negative for both limiting cases considered above by similar reasoning. However, the intermediate α between these two limits cannot be analysed in a simple way. The detail and formal proof of the result can be found in the 'Method' section, where it is shown that ∂ g S α ( g ) still remains negative for all α >0. Thus, differential local convertibility exists in this phase. These results indicate that at the critical point, there is a distinct change in the nature of the ground state. Before the critical point, a small perturbation of the external magnetic field results in a change of the ground state that cannot be implemented without two-body quantum gates. In contrast, after phase transition, any such perturbation may be simulated completely by LOCC. XY model We generalize our analysis to the XY model, with Hamiltonian for different fixed values of γ >0. The transverse Ising model thus corresponds to the the special case for this general class of models, in which γ =1. For γ ≠1, there exists additional structure of interest in phase space beyond the breaking of phase flip symmetry at g =1. In particular, there exists a circle, g 2 + γ 2 =1, on which the ground state is fully separable. The functional form of ground state correlations and entanglement are known to differ substantially on either side of the circle [22] , [23] , [24] , which motivates the perspective that the circle is a boundary between two differing phases. Indeed, such a division already exists from the perspective of an entanglement phase diagram, where different 'phases' are characterized by the presence and absence of parallel entanglement [25] . Analysis of local convertibility reveals that from the perspective of computational power under adiabatic evolution we may indeed divide the system into three separate phases ( Fig. 3 ). While the disordered paramagnetic phase remains locally convertible, the local convertibility of the ferromagnetic phase now depends on whether g 2 + γ 2 >1. In particular, for each fixed γ >0, the system is only locally non-convertible when We summarize these results in a 'local-convertibility phase-diagram', where the ferromagnetic region is now divided into components defined by their differential local convertibility. 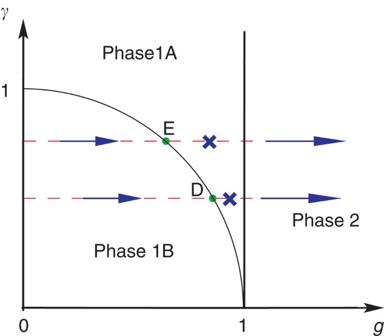Figure 3: XY model local convertibility phase diagram. Consideration of differential local convertibility separates the XY model in three phases, which we label phase 1A, phase 1B and phase 2. We consider differential local convertibility for fixed values ofγwhilegis perturbed. Differential local convertibility is featured within both phase 1B and phase 2, but not phase 1A. Figure 3: XY model local convertibility phase diagram. Consideration of differential local convertibility separates the XY model in three phases, which we label phase 1A, phase 1B and phase 2. We consider differential local convertibility for fixed values of γ while g is perturbed. Differential local convertibility is featured within both phase 1B and phase 2, but not phase 1A. Full size image Different partitions Numerical evidence strongly suggests that our results are not limited to a particular choice of bipartition. We examine the differential local convertibility when both systems of interest is partitioned in numerous other ways, where the two parties may share an unequal distribution of spins ( Fig. 4 ). The qualitative properties of ∂ g S α remain unchanged. While it is impractical to analyse all 2 N possible choices of bipartition, these results motivate the conjecture that differential local convertibility is independent of our choice of partitions. Should this be true, it has strong implications: the computation power of adiabatic evolution in different phases are drastic. In one phase, perturbation of the external field can be completely simulated by LOCC operations on individual spins, with no coherent two-spin interactions. While, in other phases, any perturbation in the external field creates coherent interactions between any chosen bipartition of the system. 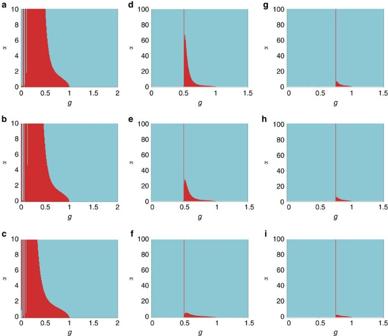Figure 4: The sign distribution of∂gSαin Ising model and XY model for different bipartitions. The sign distribution of∂gSαon the α−gplane for different bipartitions on the systems. Panels (a), (b) and (c) correspond to Ising model of sizeN=12, where Alice possesses 6,5 and 4 of the spins, respectively.∂gSαis negative in lighter regions and positive in the red regions. Clearly, regardless of choice of bipartition,∂gSαis always negative forg>1 and takes on both negative and positive values otherwise. Note that for very smallg,∂gSαonly becomes negative for very largeαand thus appears completely positive in the graph above. The existence of negative∂gSαcan be verified by analysis of∂gSαin theα→∞limit. The choice of bipartition affects only the shape of the∂gSα=0 boundary, which is physically unimportant. Panels (d), (e) and (f) correspond to XY model with fixedN=14 andL=7, 6 and 5, respectively. Panels (g), (h) and (i) correspond to XY model with fixedN=18 andL=9, 8 and 7, respectively. Here, the value ofLrepresents a bipartition in whichLqubits are placed in one bipartition andN−Lqubits in the other. The only region in which∂Sα/∂gtakes on both negative and positive values is in phase 1A. Note that the transition between phase 1A and 1B occurs atg=0.5 for(Point E inFig. 3) andg=0.75 for(Point D inFig. 3). Figure 4: The sign distribution of ∂ g S α in Ising model and XY model for different bipartitions. The sign distribution of ∂ g S α on the α− g plane for different bipartitions on the systems. Panels ( a ), ( b ) and ( c ) correspond to Ising model of size N =12, where Alice possesses 6,5 and 4 of the spins, respectively. ∂ g S α is negative in lighter regions and positive in the red regions. Clearly, regardless of choice of bipartition, ∂ g S α is always negative for g >1 and takes on both negative and positive values otherwise. Note that for very small g , ∂ g S α only becomes negative for very large α and thus appears completely positive in the graph above. The existence of negative ∂ g S α can be verified by analysis of ∂ g S α in the α → ∞ limit. The choice of bipartition affects only the shape of the ∂ g S α =0 boundary, which is physically unimportant. Panels ( d ), ( e ) and ( f ) correspond to XY model with fixed N =14 and L =7, 6 and 5, respectively. Panels ( g ), ( h ) and ( i ) correspond to XY model with fixed N =18 and L =9, 8 and 7, respectively. Here, the value of L represents a bipartition in which L qubits are placed in one bipartition and N − L qubits in the other. The only region in which ∂S α / ∂g takes on both negative and positive values is in phase 1A. Note that the transition between phase 1A and 1B occurs at g =0.5 for (Point E in Fig. 3 ) and g =0.75 for (Point D in Fig. 3 ). Full size image The study of differential local convertibility of the ground state gives direct operational significance to phase transitions in the context of quantum information processing. For example, adiabatic quantum computation (AQC) involves the adiabatic evolution of the ground state of some Hamiltonian, which features a parameter that varies with time [26] , [27] . This is instantly reminiscent of our study, which observes what computational processes are required to simulate the adiabatic evolution of the ground state under variance of an external parameter in different quantum phases. Specifically, AQC involves a system with Hamiltonian (1− s ) H 0 + sH p , where the ground state of H 0 is simple to prepare and the ground state of H p solves a desired computational problem. Computing the solution then involves a gradual increment of the parameter s . By the adiabatic theorem, we arrive at our desired solution provided the s is varied slowly enough such that the system remains in its ground state [26] , [27] . We can regard this process of computation from the perspective of local convertibility and phase transitions. Should the system lie in a phase where local convertibility exists, the increment of s may be simulated by LOCC. Thus, AQC cannot have any computational advantages over classical computation. Only in phases where no local convertibility exists can AQC have the potential to surpass classical computation. Thus, a quantum phase transition could be regarded as an indicator from which AQC becomes useful. In fact, the spin system studied in this paper is directly relevant to a specific AQC algorithm. The problem of '2− SAT on a Ring: Agree and Disagree' features an adiabatic evolution involving the Hamiltonian where s is slowly varied from 0 to 1 [26] , [27] . This is merely a rescaled version of the Ising chain studied here, where the phase transition occurs at s = 2/3. According to the analysis above, the AQC during the paramagnetic phase can be simulated by local manipulations or classical computations. For the period of ferromagnetic phase, we can do nothing to reduce the adiabatic procedure. In this paper, we have demonstrated that the computational power of adiabatic evolution in the XY model is dependent on which quantum phase it resides in. This surprising relation suggests that different quantum phases may not only have different physical properties but may also display different computational properties. This hints that not only are the tools of quantum information useful as alternative signatures of quantum phase transitions, but that the study of quantum phase transitions may also offer additional insight into quantum information processing. This motivates the study of the quantum phases within artificial systems that correspond directly to well-known adiabatic quantum algorithms, which may grant additional insight on how adiabatic computation relates to the physical properties of system that implements the said computation. There is much potential insight to be gained in applying the methods of analysis presented here to more complex physical systems that features more complex quantum transitions. In addition, differential local convertibility also may possess significance beyond information processing. One of the proposed indicators of a topological order involves coherent interaction between subsystems that scale with the size of the system [28] , [29] . In our picture, such an indicator could translate to the requirement for non-LOCC operations within appropriate chosen bipartite systems. Thus, differential local convertibility may serve as an additional tool for the analysis of such order. Eigenvalue properties For the transverse field Ising model, the largest eigenvalue λ 1 monotonically increases while the second λ 2 monotonically decreases for all g ( Fig. 2 ). In the thermodynamic limit, all the other eigenvalues increase in the g <1 region and decrease in the g >1 region. Moreover, the eigenvalues other than the largest two are much smaller than λ 1 and λ 2 . Therefore, we can average them when considering their contribution to the Renyi entropy. Thus, the eigenvalues are assumed to be 0.5+ δ , 0.5− ɛ , ( ɛ − δ )/(2 n −2), ( ɛ − δ )/(2 n −2),... when g <1, and 1− δ ′ − ɛ ′, ɛ ′, δ ′/(2 n −2),..., when g >1, where n is the particle number belonging to Alice and certainly Bob has the other N − n particles. Because of some obvious reasons such as λ 1 > λ 2 > λ 3 ... and all these eigenvalues are positive, and so on, we can derive the following relations easily: 0<δ< ɛ <0.5, 0<∂δ/∂ g <∂ ɛ /∂ g , 0<δ′< ɛ ′<0.5, ∂δ′/∂ g <0, and ∂ɛ ′/ ∂g <0. Then we can prove the main result for each phase region. Namely, in the g <1 phase, ∂ g S α is positive for small α but negative for large α ; and for the g >1 phase, ∂ g S α <0 for all α . Ferromagnetic phase In the ferromagnetic phase g <1, the eigenvalues are 0.5+ δ , 0. 5− ɛ , ( ɛ − δ )/(2 n −2), ( ɛ − δ )/(2 n −2),.... So the Renyi entropy and In the thermodynamic limit N →Ŝ, ( ɛ − δ )/(2 n −2)→ 0. When When as and 0< ∂δ / ∂g < ∂ɛ / ∂g , we can see that the solution of ∂S α / ∂g =0 (labelled as α 0 ) always exists in the region and ∂S α / ∂g will be negative as long as α > α 0 . Moreover, we can also see that the smaller g is, the smaller δ and ɛ are, and the smaller (1+( ɛ + δ )/(0.5− ɛ )) is, and therefore the larger α 0 should be. This explains why we need to examine larger value of α to find the crossing when g is very small. Notice that in the above analysis, we used the N →∞ condition in the g <1 region. We can also find that in Fig. 4 for finite N =12 there is some small green area in the region However, in the above analysis of infinite N , this area should be totally red. This difference is owing to the finite size effect. Paramagnetic phase In the paramagnetic phase, g >1. The eigenvalues are 1− δ ′− ɛ ′, ɛ ′, δ ′/(2 n −2),.... The Rényi entropy And where ∂δ ′/ ∂g , ∂ɛ ′/ ∂g <0; and ɛ ′/(1− ɛ ′− δ ′), δ ′/(1− ɛ ′− δ ′)(2 n −2) ∈ (0,1), as λ 1 > λ 2 > λ 3 . So when α >1, [(...) α−1 −1]<0, {...}>0, α /(1− α )<0. We have ∂S α / ∂g <0; and when 0< α <1, [(...) α−1 −1]>0, {...}<0, α /(1− α )>0. We also have ∂S α / ∂g <0. Hence, we can obtain that when g >1, ∂S α / ∂g <0 for all α >0. If we consider the full condition for the local convertibility, which includes the generalization of α to negative value, it also can be proved easily that the local convertible condition ∂ g S α / α >0 for all α is satisfied in the g >1 phase. As for the g <1 phase, the sign changing in the positive α already violates the local convertible condition, so that we do not need to consider the negative α part. In fact, generally speaking, for the study of differential local convertibility, we can only focus on the positive α part, because the derivative of Rényi entropy over the phase transition parameter will necessarily generate a common factor α , which will cancel the same α in the denominator. To conclude, In the g >1 phase ∂S α / ∂g is negative for all α , and in the region it is positive, while in the region it can be either negative or positive with the boundary depending on the solution of equation (4). How to cite this article: Cui, J. et al . Quantum phases with differing computational power. Nat. Commun. 3:812 doi: 10.1038/ncomms1809 (2012).